New materials for methane capture from dilute and medium-concentration sources Methane (CH 4 ) is an important greenhouse gas, second only to CO 2 , and is emitted into the atmosphere at different concentrations from a variety of sources. However, unlike CO 2 , which has a quadrupole moment and can be captured both physically and chemically in a variety of solvents and porous solids, methane is completely non-polar and interacts very weakly with most materials. Thus, methane capture poses a challenge that can only be addressed through extensive material screening and ingenious molecular-level designs. Here we report systematic in silico studies on the methane capture effectiveness of two different materials systems, that is, liquid solvents (including ionic liquids) and nanoporous zeolites. Although none of the liquid solvents appears effective as methane sorbents, systematic screening of over 87,000 zeolite structures led to the discovery of a handful of candidates that have sufficient methane sorption capacity as well as appropriate CH 4 /CO 2 and/or CH 4 /N 2 selectivity to be technologically promising. Methane (CH 4 ) is a substantial driver of global climate change, contributing 30% of current net climate forcing [1] . In addition, concern over methane is mounting due to leaks associated with rapidly expanding unconventional oil and gas extraction and the potential for large-scale release of methane from the Arctic [2] . At the same time, methane is a growing source of energy [3] , and aggressive methane mitigation is increasingly recognized as a key to avoiding dangerous levels of global warming [4] , [5] . Methane is emitted at a wide range of concentrations from a variety of sources, including natural gas systems, enteric fermentation (livestock), landfills, coal mining, manure management, wastewater treatment, rice cultivation and a few combustion processes. We can generally group the methane concentrations of sources into three categories: high purity (>90%), medium purity (5–75%) and dilute (<5%). High-purity methane can be sold to the commodity natural gas market or converted to other chemicals (for example, methanol and carbon black) by current industrial practices. Medium-purity methane includes landfill gas, coal-mine drainage gas, anaerobic digester gas and low-quality gas from fossil formations. A variety of technologies has been developed for generating electricity or high-grade process heat from medium-purity methane, including technologies such as the homogeneous charge gas engine that operates just above the methane flammability limit in air (5%). Small or inconvenient flows of medium-purity methane are often simply flared [2] . Treatable dilute methane sources are some of the largest in total emissions, including coal-mine ventilation air, manure storage headspace and animal feeding house ventilation air. Some technologies have been developed for oxidizing dilute methane, such as the thermal flow-reversal reactor, but they generally yield only low-grade heat or small amounts of electricity as a co-benefit. It is highly desirable to be able to concentrate a dilute methane stream to medium purity to effectively utilize the energy, or to concentrate a medium-purity stream to high purity to convert it to a liquid or sell it. Conversion is especially attractive for many small or remote sources. Purification of some medium and higher-purity natural gases is currently practiced industrially by sorption of the non-methane components (CO 2 and H 2 S). The practice becomes uneconomic or impractical below about 40% methane [6] . For methane concentrations <40%, or for separation of methane from air rather than acid gases, we would like a sorbent for methane itself. In this contribution, we explore the possibility of using a sorbent for methane purification. We consider the following general problems: (1) concentrating a medium-purity stream to the high-purity range and (2) concentrating a dilute stream to the medium-purity range. For purposes of analysis, our proxies for these cases are (1) a low-quality natural gas (simplified as 30% CH 4 and 70% CO 2 by mole fraction at a total pressure of 70 bar) and (2) coal-mine ventilation air (simplified as 1% CH 4 , 1% CO 2 and 98% N 2 at a total pressure of 1 bar). Both of these are potential large-scale, high-impact applications for a sorbent for methane. The example cases illustrate two general characteristics of methane purification. First, because processes related to the ones that produce methane also produce CO 2 , almost all natural methane streams contain significant levels of CO 2 . Second, for dilute streams, N 2 is the dominant component to exclude. O 2 is also abundant, but for combustion applications, it is desirable to carry at least as much O 2 as CH 4 through the process. For going from medium- to high-purity methane, a sorbent selectivity of CH 4 over CO 2 greater than 1 is required and generally, the higher the selectivity, the fewer absorption–desorption cycles required to reach desired purity. For going from dilute to medium purity, the selectivity of CH 4 over N 2 is more important for determining the number of cycles. The selectivity of CH 4 over CO 2 may also be important, depending on the application. For combustion at low concentrations (e.g., 5% CH 4 ), selectivity is not relevant. However, if the gas is to be further purified, or is to be used in an advanced (e.g., biologically based) conversion process, then selectivity close to or greater than 1 is desirable. In this contribution, we carry out thorough exploration of two different classes of capture materials for their effectiveness in methane capture: (1) liquid solvents and (2) nanoporous zeolites. We show that although none of the common solvents (including ionic liquids (ILs)) appears to possess enough affinity towards methane to be of practical use, systematic screening of around one hundred thousand zeolite structures has uncovered a few nanoporous candidates that appear technologically promising. We use free-energy profiling and geometric analysis in these candidate zeolites to understand how the distribution and connectivity of pore structures and binding sites can lead to enhanced sorption of methane while being competitive with CO 2 sorption at the same time. Liquid solvents for methane capture Liquids have traditionally been known as poor absorbers of methane, however, the experimental literature has limited data for methane solubility both in conventional solvents as well as in ILs. A thorough investigation of liquid solvents is important for two reasons: (1) a good liquid solvent for methane could not only be used as a capture agent but also could be injected to break down methane hydrate (clathrate), and extract methane from this potentially huge untapped energy source [7] , [8] , [9] and (2) there have been recent experimental attempts of exploring novel solvents (ILs) for efficient absorption [10] and catalytic conversion [11] of methane; a systematic in silico study could contribute greatly to such progress. To compute methane solubility in liquids, we adopted an implicit solvent method, that is, COSMO-RS [12] , [13] , in which one represents both the solute and solvent molecules by the histogram of their surface screening charges called the σ-profile. All interactions, including Coulombic, van der Waals and hydrogen-bond interactions, are then defined in terms of these σ-profiles. One can use this formalism to compute the partition function, the Gibbs free energy and many other thermodynamic quantities, including pseudo-chemical potentials ( μ *) [14] . The pseudo-chemical potential of any solute present in x mole fraction in a solution ( μ solvent *) is defined as its chemical potential ( μ ) without the ideal entropy of mixing term k B T ln( x ); in other words, μ = μ solvent *+ k B T ln( x ). μ self * is the pseudo-chemical potential of the solute in its own pure liquid state ( x =1), where the chemical potential is μ = μ self *+ k B T ln(1)= μ self *. Mole-fraction solubility ( x ) can be computed by equating the two chemical potentials, μ solvent *+ k B T ln( x )= μ self *, which leads to the following equation: Note that by its very definition the pseudo-chemical potential includes a contribution from the activity coefficient, which, however, becomes negligible in the limit of infinite dilution. When the solute is dissolving from the gas phase, one needs to relate the quantity μ * self to the chemical potential in the gas phase, which can be expressed as a function of the gas fugacity [15] . However, because our liquid exploration involved a fixed pressure (1 bar) and a fixed temperature (300 K), we found it more convenient to use μ * self as a fitting parameter so as to match the experimental solubility of all relevant gases, that is, CH 4 (refs 9 , 16 ), N 2 (refs 17 , 18 ) and CO 2 (ref. 19 ) in one specific standard solvent, that is, ethanol. This led to the values of μ * self =−26.8, −27.6 and −17.6 kJ mol −1 for CH 4 , N 2 and CO 2, respectively, to be used with COSMO-RS-computed μ solvent under the parameter settings described in the Methods section. First, we explored the feasibility of using liquid solvents to concentrate coal-mine ventilation air, represented by (in mole fraction) 1% CH 4 , 1% CO 2 and 98% N 2 at a total pressure of 1 bar. The aim was to create an output stream with >5% CH 4 . This translates to a desired CH 4 /N 2 selectivity >5. Here we define selectivity as the ratio of Henry’s constants, for example, CH 4 /N 2 selectivity= K H (CH 4 )/ K H (N 2 ). Roughly speaking, a CH 4 /N 2 selectivity of ~5 (along with CO 2 /CH 4 selectivity not much larger than 1) leads to an output stream of 5% CH 4 within one cycle (because the starting concentration of CH 4 ~1%). The actual CH 4 concentration in the output stream will depend on the number of stages and other processing parameters. However, for economic reasons, the idea is to look for materials that can lead to the desired CH 4 concentration in as little cycles as possible. The presence of O 2 was not considered explicitly just for simplicity, and it was assumed that the output stream will have sufficient O 2 to be able to combust the methane. For some applications (further purification of the gas or some chemical conversions), we require CH 4 /CO 2 selectivity to be not much less than 1 as otherwise, CO 2 becomes the major fraction in the output stream. With this in mind, we computed the solubilities (using equation (1)) of CH 4 , N 2 and CO 2 in 73 common room-temperature liquid solvents at T =300 K and P =1 bar, which also include 10 common ILs (see Supplementary Table S1 ). The conventional solvents were chosen from a wide variety of classes, including alkanes, cyclo-alkanes, alkenes, alkynes, aromatics, alcohols, aldehydes, ether, ketones, amines and thiols. 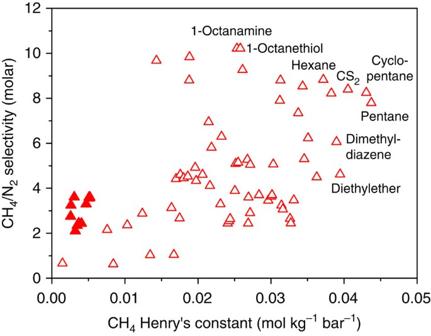Figure 1: CH4/N2molar selectivity versus CH4Henry’s constant in liquid solvents. Selectivity is defined as the ratio of Henry’s constantsKH(CH4)/KH(N2). Results are shown for 73 common liquid solvents (including 10 ILs). All calculations were performed atT=300 K andP=1 bar. The names of the most interesting solvents are indicated. The ILs are indicated by filled symbols. The full solvent list is provided inSupplementary Table S1. Figure 1 plots the CH 4 /N 2 selectivity (defined as the ratio of Henry’s constants K H (CH 4 )/ K H (N 2 )) on the y axis and the corresponding CH 4 Henry’s constant ( K H (CH 4 ) in mol kg −1 bar −1 ) on the x axis. In general, the solubility in the ILs is relatively low in the relevant conditions such that one can reliably compute selectivity from the ratio of Henry’s constants. Interestingly, there are many solvents with CH 4 /N 2 selectivity >5, with 1-octanamine and 1-octanethiol having values >10. The solvents with the highest CH 4 solubility (that is, highest K H (CH 4 )) appear to be the small alkanes like pentane, cyclo-pentane, hexane and so on, as well as carbon disulphide (CS 2 ). All of these solvents also have desirable CH 4 /N 2 selectivity values of ~8. Unfortunately, the Henry’s constant is too low, being ~0.044 mol kg −1 bar −1 even for the best solvent, that is, pentane. For an inlet partial methane pressure of 0.01 bar, this would amount to a loading of only 4.4 × 10 −4 mol kg −1 , which does not make it economically viable. In addition, Fig. 2 shows that even for the alkanes the highest value of the CH 4 /CO 2 selectivity is low, being only 0.36 for cyclo-decane and 0.34 for pentane. This means that in the output stream there will be roughly three times more CO 2 as compared to CH 4 . Figure 1: CH 4 /N 2 molar selectivity versus CH 4 Henry’s constant in liquid solvents. Selectivity is defined as the ratio of Henry’s constants K H (CH 4 )/ K H (N 2 ). Results are shown for 73 common liquid solvents (including 10 ILs). All calculations were performed at T =300 K and P =1 bar. The names of the most interesting solvents are indicated. The ILs are indicated by filled symbols. The full solvent list is provided in Supplementary Table S1 . 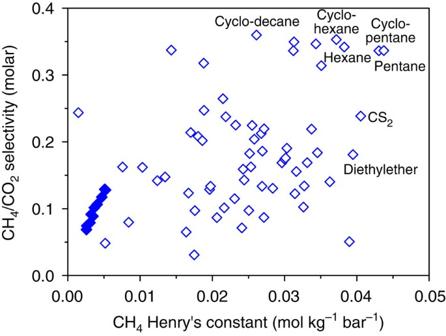Figure 2: CH4/CO2molar selectivity versus CH4Henry’s constant in liquid solvents. Selectivity is defined as the ratio of Henry’s constantsKH(CH4)/KH(CO2). Results are shown for 73 common liquid solvents (including 10 ILs). All calculations were performed atT=300 K andP=1 bar. The names of the most interesting solvents are indicated. The ILs are indicated by filled symbols. The full solvent list is provided inSupplementary Table S1. Full size image Figure 2: CH 4 /CO 2 molar selectivity versus CH 4 Henry’s constant in liquid solvents. Selectivity is defined as the ratio of Henry’s constants K H (CH 4 )/ K H (CO 2 ). Results are shown for 73 common liquid solvents (including 10 ILs). All calculations were performed at T =300 K and P =1 bar. The names of the most interesting solvents are indicated. The ILs are indicated by filled symbols. The full solvent list is provided in Supplementary Table S1 . Full size image The 10 ILs screened in Figures 1 and 2 (filled symbols) include cationic classes imidazolium, ammonium, phosphonium and pyridinium, and anions BF 4 , PF 6 and Tf 2 N (refs 15 , 20 ). We find that the highest CH 4 solubility in these classes of ILs occurs in the [ammonium][Tf 2 N] systems with a Henry’s constant of 0.005 mol kg −1 bar −1 or less, that is, almost an order of magnitude smaller than that in pentane. This is consistent with the limited available experimental data [10] , [21] . The CH 4 /CO 2 selectivity in ILs is also much worse than regular alkanes, being typically <0.15, which might be expected, given the ionic environment. The above analysis clearly demonstrates that liquid solvents, including ILs, are not suitable for concentrating and utilizing methane from low to medium emission sources—the methane solubility is too low, and the CH 4 /CO 2 selectivity is not favourable. Thus, we turned to another system with a large number of possible structural and compositional varieties, that is, nanoporous solids, like zeolites. Zeolites for methane capture Zeolites are porous materials commonly used as adsorbents. Because of their diverse topology resulting from various networks of the framework atoms, zeolites can be used for many different types of gas separations and storage applications. In this work, we analysed 190 experimentally realized International Zeolite Association (IZA) structures and over 87,000 predicted crystallography open database (PCOD) structures from Deem’s hypothetical zeolite database [22] to search for materials suitable for methane capture. Because of the quadruple moment of CO 2 , the interaction between the CO 2 molecules and the framework atoms are generally much stronger than for the CH 4 molecules. Accordingly, finding zeolite structures that simultaneously lead to a large adsorbed CH 4 concentration (relative to adsorbed CO 2 ) and high CH 4 loading poses a significant challenge even with the large number of diverse zeolite structures at our disposal. For mixtures that contain methane at relatively low pressure, the binding energy of methane is the primary factor that determines the performance of the structure. On the other hand, for separations that occur at higher pressures, the CH 4 –CH 4 interaction could also play a significant role. Thus, we expect that the total pressure of the initial mixture gas will largely dictate the type of materials optimal for methane capture. 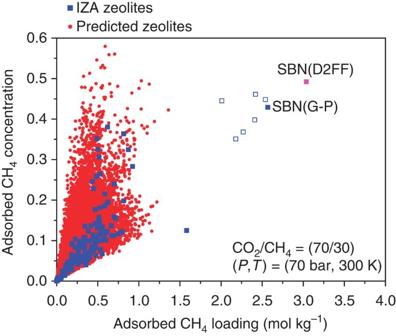Figure 3: Molar concentration of CH4in the adsorbed phase versus CH4loading in zeolites. Results are shown for 190 IZA (blue) and over 87,000 predicted (red) zeolite structures with input gas-phase mixture composition of 30% CO2and 70% CH4at pressure of 70 bar andT=300 K. The SBN that shows exceptional performance for this separation is plotted for two different force fields, Garcia-Perez (blue—solid) and D2FF (pink—solid). The unit cells of the SBN were changed from −3 to 3% of their original sizes, and relaxed using DFT for Garcia-Perez (blue—no fill). First, we performed the zeolite screening for the application involving a low-quality natural gas mixture feed consisting of 30% CH 4 and 70% CO 2 (in mole fraction) at 70 bar and 300 K. Figure 3 indicates the adsorbed CH 4 concentration (mole fraction) in the adsorbed gas mixture as a function of the adsorbed amount of CH 4 (that is, CH 4 loading) for all of the IZA and the predicted zeolite structures. The results immediately reveal an IZA structure, SBN, that stands out in its performance—roughly 2.75 (mol kg −1 ) adsorbed CH 4 and 45% adsorbed CH 4 concentration. We also utilized the recently published force field D2FF, which is developed based on dispersion-corrected density functional theory (DFT), from Sholl and co-workers [23] to compute the SBN CO 2 adsorption isotherms. Adsorption isotherms calculated via D2FF have been shown to accurately reproduce the experimental isotherms for CHA, MFI and DDR silicate zeolite structures [23] . In our work, the SBN CO 2 isotherms obtained from D2FF predict even better overall performance (see Fig. 3 ) with reduced CO 2 uptake for all of the pressure values. To further test the robustness of our finding, sensitivity analysis was conducted by changing (in steps of 1%) the SBN lattice parameters from −3 to +3% of the original optimized value of a =14.37 Å, b =12.45 Å and c =13.85 Å. For each perturbed structure, the lattice constants were kept fixed while the atomic coordinates were optimized using DFT with the quantum code SIESTA (ref. 24 ). As shown in Fig. 3 , all of the perturbed SBN data points are close to the original SBN data, indicating that in spite of a small dependence of its performance on force field parameters and lattice constant, SBN is clearly one of the best structures for methane capture. Figure 3: Molar concentration of CH 4 in the adsorbed phase versus CH 4 loading in zeolites. Results are shown for 190 IZA (blue) and over 87,000 predicted (red) zeolite structures with input gas-phase mixture composition of 30% CO 2 and 70% CH 4 at pressure of 70 bar and T =300 K. The SBN that shows exceptional performance for this separation is plotted for two different force fields, Garcia-Perez (blue—solid) and D2FF (pink—solid). The unit cells of the SBN were changed from −3 to 3% of their original sizes, and relaxed using DFT for Garcia-Perez (blue—no fill). Full size image To further explore the reason behind the exceptional performance of SBN, we plot in Fig. 4 the simulated adsorption isotherm curves and the free-energy landscapes in this zeolite for both CO 2 and CH 4 . Within the idealized SBN structure, blue represents low-energy regions and red represents high-energy regions, with the rest indicating inaccessible regions. To help with the analysis, the adsorption isotherm curves are divided into three regimes based on the total pressure (that is, P <1 bar, 1 bar< P <100 bar and P >100 bar), representing the Henry regime, strong CH 4 –CH 4 interaction regime and saturation regime, respectively (see Fig. 4 ). In the Henry regime ( P <1 bar), the guest particle–framework interaction dominates the adsorption properties where the Henry’s constant K H =0.86 and 0.52 mol kg −1 bar −1 for CO 2 and CH 4 , respectively, leading to higher uptake of CO 2 in this region. The difference can be explained by comparing the binding energy values (CH 4 : −22.09 kJ mol −1 and CO 2 : −28.57 kJ mol −1 ) of the two molecules. At P ~5 bar, the two isotherm curves intersect each other, beyond which the CH 4 uptake becomes larger. To understand the increased uptake of CH 4 in SBN at P >5 bar, we analyse in Fig. 4 the free-energy profiles of CO 2 and CH 4 . We find that the CH 4 adsorption sites are highly localized with each site connected to three nearest neighbour adsorption sites (indicated by yellow arrows in Fig. 4 ) with a separation barrier. The distances between these adsorption sites range from 4 to 4.6 Å with the average being at around 4.33 Å. Such separation values align closely with the minimum energy distance of two centre-of-mass CH 4 molecules, ~4.2 Å. On the other hand, the adsorption sites for CO 2 are less distinct from one another, and do not in general correspond to optimal CO 2 –CO 2 distances. As a result, the CH 4 uptake in SBN is higher than that of CO 2 uptake for P up to a few thousand bars, well above the pressures considered for low-quality natural gas separations. At P ≥100 bar, the CH 4 loading saturates to 16 molecules per unit cell, equal to the number of distinct CH 4 adsorption sites that can be counted from the free-energy profile in Fig. 4 . 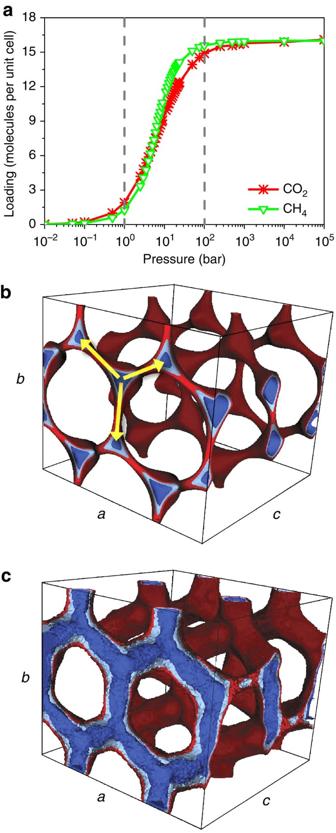Figure 4: Zeolite SBN CO2/CH4adsorption isotherm curves and unit-cell free-energy profiles. (a) CO2(red) and CH4(green) adsorption isotherm data atT=300 K where the two curves intersect one another atP=5 bar andP=105bar. The dashed lines divide the isotherms into three important regions: (1) Henry regime, (2) strong CH4–CH4interaction regime and (3) saturation regime. Free-energy landscape inside SBN unit cell for (b) CH4and (c) CO2molecule with lattice parametersa=14.374 Å,b=12.448 Å andc=13.846 Å. Dark blue represents low-energy strong binding sites, and red represents high energies. The three yellow arrows separate one binding site to another, and the distance values range from 4 to 4.6 Å. Figure 4: Zeolite SBN CO 2 /CH 4 adsorption isotherm curves and unit-cell free-energy profiles. ( a ) CO 2 (red) and CH 4 (green) adsorption isotherm data at T =300 K where the two curves intersect one another at P =5 bar and P =10 5 bar. The dashed lines divide the isotherms into three important regions: (1) Henry regime, (2) strong CH 4 –CH 4 interaction regime and (3) saturation regime. Free-energy landscape inside SBN unit cell for ( b ) CH 4 and ( c ) CO 2 molecule with lattice parameters a =14.374 Å, b =12.448 Å and c =13.846 Å. Dark blue represents low-energy strong binding sites, and red represents high energies. The three yellow arrows separate one binding site to another, and the distance values range from 4 to 4.6 Å. Full size image For coal-mine ventilation air comprised of 1% CH 4 , 1% CO 2 and 98% N 2 at a total pressure of 1 bar, similar analysis was conducted to evaluate structures suitable for this separation. The three-component Ideal Adsorbed Solution Theory was utilized to obtain the mixture loading values from the pure component isotherms. 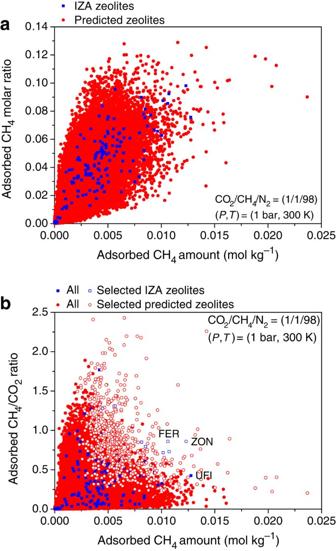Figure 5:CH4capture using zeolites for coal-mine ventilated air. (a) Adsorbed CH4concentration as function of CH4loading for IZA (blue) and predicted (PCOD) (red) structures. (b) The same data points are plotted with adsorbed CH4/CO2ratio as a function of adsorbed CH4amount. The ‘no fill’ data points represent zeolite structures fromathat have adsorbed CH4molar ratio >0.08. Thus, the best structures are structures within the set of ‘no fill’ data points that also have large adsorbed CH4amount and large CH4/CO2ratio values. Figure 5a shows the results for the IZA and the predicted zeolite structures. At this condition, the uptake values of these three gases tend to lie within the linear region in the pure component isotherms for most zeolite structures, and accordingly, a strong correlation exists between Henry’s constant and uptake values at this pressure. Thus, it is not surprising that in our analysis, we found that the top 20 structures (where the metric was taken to be simply the product of the solubility and selectivity) in the predicted zeolite database possess a CH 4 Henry’s constant >1.36 mol kg −1 bar −1 at 300 K, which puts them within the top 0.1% of the largest K H in the database. Zeolite SBN, which has a relatively smaller K H =0.52 mol kg −1 bar −1 , is predicted to have poor performance for this separation. The analysis of the free-energy landscape reveals that most of the top structures are comprised of one-dimensional channels for the CH 4 molecules. In addition, geometry analysis utilizing Zeo++ [25] indicates that the maximum included sphere along these free paths has diameters between 5–6 Å. Thus, these channels can be characterized as narrow and not cage-like. In general, the zeolite structures with narrow channels can form strong CH 4 binding sites as the number of framework oxygen atoms located within close (i.e., 3–4 Å) vicinity to the centre of the binding sites can be maximized within this topology. On the other hand, a cage-like environment tends to provide fewer framework oxygen atoms at optimum distances from the CH 4 , and thereby leads to low Henry’s constant values. Figure 5: CH 4 capture using zeolites for coal-mine ventilated air. ( a ) Adsorbed CH 4 concentration as function of CH 4 loading for IZA (blue) and predicted (PCOD) (red) structures. ( b ) The same data points are plotted with adsorbed CH 4 /CO 2 ratio as a function of adsorbed CH 4 amount. The ‘no fill’ data points represent zeolite structures from a that have adsorbed CH 4 molar ratio >0.08. Thus, the best structures are structures within the set of ‘no fill’ data points that also have large adsorbed CH 4 amount and large CH 4 /CO 2 ratio values. Full size image In this separation, we further focused on zeolite structures that also possess high adsorbed CH 4 /CO 2 ratio. For this low-pressure condition, the adsorbed CH 4 /CO 2 ratio can be regarded as the previously defined selectivity as the ratio of Henry’s constants. Figure 5b shows the CH 4 /CO 2 selectivity of all structures plotted in Fig. 5a as a function of adsorbed CH 4 amount, with open symbols indicating the structures with adsorbed CH 4 molar ratio >0.08 in Fig. 5a . The IZA structures with the largest adsorbed CH 4 /CO 2 ratio were identified to be ZON and FER, with K H (CH 4 )=1.29 and 1.12 mol kg −1 bar −1 , respectively. Moreover, we have identified many PCOD structures that have a very large adsorbed CH 4 /CO 2 ratio (>2.00), which can be promising for the separation (e.g., PCOD8301873 and PCOD8307399). Although IZA structures such as UFI have even larger K H (CH 4 )=1.39 mol kg −1 bar −1 than what is computed for ZON and FER, the CH 4 /CO 2 selectivity is only 0.44, which is much smaller compared to ZON (0.85) and FER (0.94). Analysis of these three structures based on the free-energy profiles reveals that the number of low-energy adsorption sites for CO 2 is larger compared with CH 4 , which might partially be responsible for the relatively low CH 4 /CO 2 selectivity value in UFI. In general, it is difficult to find common characteristics among zeolite structures that possess both large K H (CH 4 ) and large CH 4 /CO 2 selectivity as intricate and subtle differences in the framework composition seem to make large contributions. With the aim of discovering materials capable of isolating or concentrating methane at minimum energy costs, we have carried out extensive in silico screening of a large number of conventional liquids and ILs, as well as over 87,000 zeolite structures. Cutting-edge computational tools were employed, including a DFT-based quantum-chemical implicit solvent formalism [13] for the liquid solvents and a recently developed, highly efficient sorption code [26] , [27] for the zeolites that employs classical force fields with well-validated parameter sets. Two specific application areas were targeted, that is, concentrating methane from a medium-concentration source to a high concentration (for example, purifying a low-quality natural gas) and concentrating a very dilute methane stream into one of the moderate concentrations (for example, enabling energy production from coal-mine ventilation air). Both these applications warrant materials that need to have higher affinity to methane than to CO 2 , a challenging proposition given methane's essentially non-polar character. In this regard, all the liquids in our investigation fall short—the best overall liquid, pentane, has the required CH 4 /N 2 selectivity (~8), but low Henry’s constant (0.044 mol kg −1 bar −1 ) and low CH 4 /CO 2 selectivity (0.34). However, some of the zeolites show considerable promise both in terms of CH 4 uptake capacity and CH 4 /CO 2 selectivity. Particularly noteworthy is the zeolite SBN, which has a large number of binding sites that are formed in such a way that maximizes the CH 4 –CH 4 interactions, resulting in extraordinarily high performance for concentrating methane from a medium-concentration source to a high concentration. For dilute methane, on the other hand, there are zeolites like ZON and FER that possess large K H (CH 4 ) as well as high CH 4 /CO 2 selectivity, making them excellent candidates for concentrating dilute methane stream into moderate concentration. For the latter separation, we have also identified other structures in the predicted zeolite database that could potentially outperform ZON and FER. All these structures consist of narrow one-dimensional channels that create strong binding sites for CH 4 by having a significant number of framework oxygen atoms at optimal distances from the CH 4 centre. For further information about these IZA zeolite structures (e.g. lattice constant, atomic positions and space group), please refer to http://www.iza-structure.org/databases/ . Besides pure silica zeolite structures, we have also conducted large-scale screening on aluminosilicate zeolite structures in which some of the silicon atoms are substituted with aluminium atoms with the addition of cations to ensure charge neutrality. Similar work has been conducted in the past to analyse CO 2 adsorption in aluminosilicate zeolite structures [28] . In our analysis, we found aluminosilicate zeolite structures to be, in general, sub-optimal for methane reduction; the presence of cations creates strong binding sites for the CO 2 molecule, and subsequently leads to inferior CH 4 /CO 2 selectivity values. However, more in-depth study needs to be conducted to determine whether we can completely rule out aluminosilicate zeolites as a viable class of materials for methane capture. One can also attempt to screen a large database of porous materials such as metal-organic frameworks, zeolitic imidazolate frameworks or covalent organic frameworks [29] to identify structures optimal for methane capture. Unfortunately, many of the synthesized structures possess strong interactions between the metal atoms and the CO 2 molecules, and thus are more promising for CO 2 capture. Finally, there have been recent attempts in the literature to utilize activated carbon [30] and graphene [31] for methane capture. Activated carbon could be a good storage medium for relative pure methane [30] , but is probably not an ideal system to preferentially adsorb CH 4 over CO 2 . Graphene, with proper doping and inter-layer spacing could potentially isolate CH 4 (ref. 31 ), but more work needs to be done to optimize such a system for selective methane capture with high loading capacity. A large-scale screening approach such as ours could be appropriate for such an exploration. Solubility calculations in liquid solvents and ILs As in our previous work [32] , the surface screening charges (and the corresponding σ-profiles) were computed using the DFT code Turbomole [33] , the Becke–Perdew exchange-correlation functional [34] , [35] and an all-electron representation using the triple-zeta valence basis set with polarization [36] , [37] . These σ-profiles were then used to compute the pseudo-chemical potentials μ solvent * using the commercial COSMO-RS code COSMOTherm (version C2.1, Release 01.10), available from Cosmologic Inc. ( http://www.cosmologic.de ). For an IL, a separate σ-profile is constructed for the cation and the anion, and the solvent represented as a 50:50 molar mixture of the two fragments. From extensive tests on the aqueous solubility of a large data set of drug molecules or organic solutes, it appears that COSMO-RS incurs an average error of the order of 0.3–0.5 log units [38] . Based on the above, an accuracy of the computed solubility to within a factor of 2–3 can be considered reasonable. Calculation of adsorption isotherms in zeolites The Henry’s constant and the pure component adsorption isotherms for CO 2 , CH 4 and N 2 gas molecules were computed using our highly efficient graphics processing unit code [26] , [27] , and the Ideal Adsorbed Solution Theory was then applied to estimate the mixture component uptake to reproduce the aforementioned conditions relevant to methane separations [39] . In our simulations, all interactions between gas molecules and the zeolite framework were described at the classical force field level with atomic partial charges (for Coulombic interactions) and 12-6 Lennard–Jones parameters (for van der Waals interactions) taken from Garcia-Perez et al . [40] The framework was assumed to be rigid throughout the simulations, an assumption that is considered to be reasonable in zeolite structures [41] . How to cite this article: Kim, J. et al . New materials for methane capture from dilute and medium-concentration sources. Nat. Commun. 4:1694 doi: 10.1038/ncomms2697 (2013).